Berberine activates thermogenesis in white and brown adipose tissue Obesity develops when energy intake exceeds energy expenditure. Promoting brown adipose tissue formation and function increases energy expenditure and hence may counteract obesity. Berberine (BBR) is a compound derived from the Chinese medicinal plant Coptis chinensis . Here we show that BBR increases energy expenditure, limits weight gain, improves cold tolerance and enhances brown adipose tissue (BAT) activity in obese db/db mice. BBR markedly induces the development of brown-like adipocytes in inguinal, but not epididymal adipose depots. BBR also increases expression of UCP1 and other thermogenic genes in white and BAT and primary adipocytes via a mechanism involving AMPK and PGC-1α. BBR treatment also inhibits AMPK activity in the hypothalamus, but genetic activation of AMPK in the ventromedial nucleus of the hypothalamus does not prevent BBR-induced weight loss and activation of the thermogenic programme. Our findings establish a role for BBR in regulating organismal energy balance, which may have potential therapeutic implications for the treatment of obesity. Obesity has reached epidemic proportions worldwide, leading to the development of many common medical conditions, such as type 2 diabetes and metabolic syndrome with high increasing rate, accelerated cardiovascular diseases and increased cancer risk [1] . Obesity develops when the energy intake exceeds the energy expenditure. Because the laws of thermodynamics must be obeyed, any treatment for obesity must either reduce energy intake, or increase energy expenditure, or have an effect on both at the same time [2] . While restricting caloric intake is the first line of defence against obesity, it is a critical alternative strategy to modify the metabolic efficiency and increase the energy expenditure in key metabolic organs, such as adipose tissue [3] . Mammals possess two specialized types of adipose tissue that serve opposite functions, the white and brown adipose tissues (WAT and BAT). WAT, which is characterized by large unilocular lipid-droplets-containing white adipocytes, is an active endocrine organ that regulates diverse activities, such as insulin sensitivity [4] . BAT and WAT are morphologically and functionally different tissues, and their developmental patterns are quite distinct [5] . BAT is histologically distinct from WAT, it composes of multilocular lipid droplets and large numbers of mitochondria that contain uncoupling protein-1 (UCP1). BAT plays an active role in energy expenditure by oxidizing fatty acids that are produced by triglyceride hydrolysis to generate heat [6] . BAT is a specialized tissue that dissipates chemical energy to protect against hypothermia and obesity through a process termed nonshivering thermogenesis. Clusters of UCP1-expressing multilocular adipocytes with thermogenic capacity develop in WAT in response to various stimuli, and these adipocytes have been named beige or ‘brite’ (brown in white) [7] , [8] . BAT was thought to function primarily in rodents and in newborn babies as a mechanism for facilitating the adaptation to a cold environment. Recent studies have revealed that adult humans also have functional BAT [9] , [10] , [11] , a finding that has fuelled speculation that the pharmacologic enhancement of BAT development and activity might be a useful strategy and a hopeful target for counteracting obesity. Active BAT burns lipids to produce heat, resulting in increased energy expenditure. Many studies have shown that changes in the BAT activity can profoundly affect body weight. Strategies that manipulate WAT to acquire BAT-like characteristics remain an alternative, but even less well-characterized, approach for enhancing energy expenditure and decreasing obesity [12] . Berberine (BBR) is a naturally occurring plant alkaloid present in many Chinese herbal medicines, commonly used for diarrhoea, and has been found to have a variety of metabolic benefits in recent years. In vivo and in vitro studies have shown that BBR can bring about improvements in metabolic disorders, such as insulin resistance and hyperlipidemia [13] , [14] , [15] , [16] . We analyze the mechanism of BBR in vitro , so as to evaluate its positive role in energy expenditure in vivo . We have demonstrated BBR could regulate a thermogenesis programme in both BAT and WAT, and these effects are AMPK/PGC-1α dependent. Our data establish BBR as having a previously unrecognized role in increasing energy expenditure, which might have a therapeutic role in the treatment of obesity. Effects of BBR on metabolic profile of obese mice The metabolic effects of BBR were evaluated by administering the compound to obese db/db mice. The mice were obviously protected from weight gain during 4 weeks of treatment ( Fig. 1a ). This result might be a consequence of inhibiting fat accumulation by BBR ( Fig. 1b ). The enzymes associated with hepatic injury or tissue breakdown were normal during the study, indicating that BBR was well-tolerated and the efficacy observed was not due to a toxic response ( Supplementary Fig. 1a ). 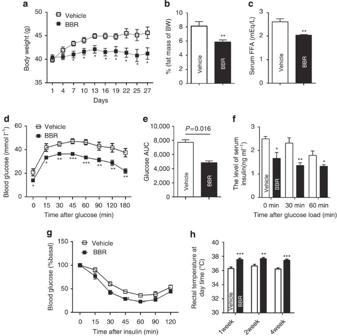Figure 1: BBR reduces obesity and improves insulin sensitivity. (a) Body weight evaluation of db/db mice treated with vehicle or BBR every 3 days (n=5). (b) Fat mass expressed as percentage of total body weight-which is shown as ratio of subcutaneous fat to body weight. (n=5). (c) Free fatty acid (FFA) levels were measured after overnight fast in the serum of mice treated with vehicle or BBR (n=5). (d) i.p. glucose tolerance test on db/db mice treated as inaand injected with 0.75 g glucose per kg after overnight fast (n=5). (e) The adjacent bar graph represents the average area under the curve (n=5). (f) Serum insulin concentration at 0 min (fasted overnight) and after glucose load at 30 and 60 min during i.p. glucose tolerance test (n=5). (g) Insulin tolerance test was evaluated throughout and injected with 1 U insulin per kg after 6 h of fasting (n=8). (h) Rectal temperature measured at 0900 hours (n=7–9). Values represent mean±s.e.m. Error bars represent s.e.m., and significant differences compared with vehicle controls are indicated by *P≪0.05, **P≪0.01 and ***P≪0.001 (assessed by Student'st-test). Figure 1: BBR reduces obesity and improves insulin sensitivity. ( a ) Body weight evaluation of db/db mice treated with vehicle or BBR every 3 days ( n =5). ( b ) Fat mass expressed as percentage of total body weight-which is shown as ratio of subcutaneous fat to body weight. ( n =5). ( c ) Free fatty acid (FFA) levels were measured after overnight fast in the serum of mice treated with vehicle or BBR ( n =5). ( d ) i.p. glucose tolerance test on db/db mice treated as in a and injected with 0.75 g glucose per kg after overnight fast ( n =5). ( e ) The adjacent bar graph represents the average area under the curve ( n =5). ( f ) Serum insulin concentration at 0 min (fasted overnight) and after glucose load at 30 and 60 min during i.p. glucose tolerance test ( n =5). ( g ) Insulin tolerance test was evaluated throughout and injected with 1 U insulin per kg after 6 h of fasting ( n =8). ( h ) Rectal temperature measured at 0900 hours ( n =7–9). Values represent mean±s.e.m. Error bars represent s.e.m., and significant differences compared with vehicle controls are indicated by * P ≪ 0.05, ** P ≪ 0.01 and *** P ≪ 0.001 (assessed by Student's t -test). Full size image Because obesity exerts detrimental actions on the plasma free fatty acid level and glucose homoeostasis, we analyzed whether BBR could normalize these parameters. Free fatty acid levels in the plasma of the BBR-treated mice were reduced ( Fig. 1c ). The mice treated with BBR had a better tolerance to a glucose load, which was particularly prominent in almost all time points of an i.p. glucose tolerance test (Fig. 1d,e ). BBR prevented the negative impact of obesity on insulin resistance; the blood insulin was also reduced after the glucose load ( Fig. 1f ). Combined with another insulin tolerance test (ITT; Fig. 1g ), these data show that BBR ameliorates glucose tolerance. Our results demonstrate that BBR reduced the body weight and improved disordered metabolic profiles. The rectal temperatures of BBR-treated animals were significantly higher than that in the vehicle group ( Fig. 1h ), which means that the mice in BBR group could generate more heat during resting periods. BBR increases energy expenditure and adaptive thermogenesis A key factor for controlling energy homoeostasis is the balance between caloric intake and energy expenditure. We analyzed the actions of BBR on energy expenditure using comprehensive lab animal monitoring system (CLAMS). When normalized to their lean mass in both the groups, the drug-treated mice showed markedly higher oxygen consumption and carbon dioxide production rates through a 12-h light/dark cycle than the control animals ( Fig. 2a–d ). The db/db mice that received BBR showed significant increases in the whole-body energy expenditure ( Fig. 2e,f ). The increase in energy expenditure in the BBR-treated mice was not due to an increase in physical activity ( Supplementary Fig. 2a ). The respiratory exchange ratio (RER) reflects the relative use of carbohydrates versus lipids as a source of energy. The RER decreased significantly upon BBR treatment, demonstrating that BBR can shift the fuel preference towards fatty acids ( Supplementary Fig. 2b ). 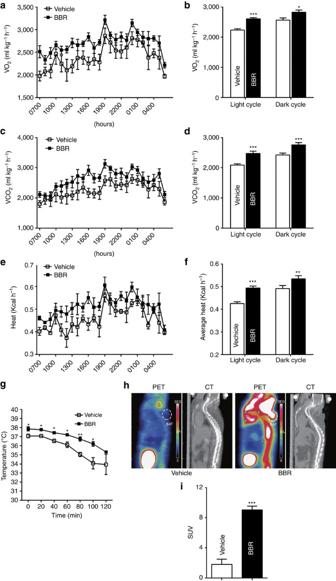Figure 2: BBR increases energy expenditure and adaptive thermogenesis. (a–f) Energy expenditure was evaluated by measurement of oxygen consumption (VO2) (a) of carbon dioxide release (VCO2) (c) over a 24 h period in db/db mice after 4 weeks of BBR treatment. Energy Expenditure expressed as Kcal h−1per animal (e) was calculated using equations described in Methods. The adjacent bar graphs represent the average for each group (bfora,dforcandffore) (n=6). (g) Body temperature during cold exposure was recorded in 20 min intervals (n=5 mice per group). After food deprivation, rectal temperatures were measured at the indicated time points for mice placed in a cold room. (h,i) PET/ CT image after injection of 18F-FDG into db/db mice treated with vehicle and BBR for 4 weeks in sagittal view (h). Anatomical site within white circle represent the interscapular BAT. Grey triangle indicated non-target absorption on those views. The activity of brown adipose tissue in grams times the mean standard uptake value (SUV) (i). Scale set, 0.1 to 3 SUV for all images. Error bars represent s.e.m., and significant differences compared with vehicle controls are indicated by *P≪0.05, **P≪0.01 and ***P≪0.001 (Student'st-test). Figure 2: BBR increases energy expenditure and adaptive thermogenesis. ( a – f ) Energy expenditure was evaluated by measurement of oxygen consumption (VO2) ( a ) of carbon dioxide release (VCO2) ( c ) over a 24 h period in db/db mice after 4 weeks of BBR treatment. Energy Expenditure expressed as Kcal h −1 per animal ( e ) was calculated using equations described in Methods. The adjacent bar graphs represent the average for each group ( b for a , d for c and f for e ) ( n =6). ( g ) Body temperature during cold exposure was recorded in 20 min intervals ( n =5 mice per group). After food deprivation, rectal temperatures were measured at the indicated time points for mice placed in a cold room. ( h , i ) PET/ CT image after injection of 18F-FDG into db/db mice treated with vehicle and BBR for 4 weeks in sagittal view ( h ). Anatomical site within white circle represent the interscapular BAT. Grey triangle indicated non-target absorption on those views. The activity of brown adipose tissue in grams times the mean standard uptake value (SUV) (i). Scale set, 0.1 to 3 SUV for all images. Error bars represent s.e.m., and significant differences compared with vehicle controls are indicated by * P ≪ 0.05, ** P ≪ 0.01 and *** P ≪ 0.001 (Student's t -test). Full size image To further examine the differences in energy expenditure among these animals, we performed a cold tolerance test to gauge adaptive thermogenesis, another major component of energy expenditure. During 2 h of exposure to cold, body temperatures of the db/db mice dropped significantly, displaying impaired thermogenesis compared with the BBR group ( Fig. 2g ). This result shows that BBR was able to increase body adaptation to cold exposure by generating more heat. BAT is a major tissue where energy is produced into the form of heat to maintain the body temperature. Active BAT can be identified in human adults by 18F-fluorodeoxyglucose (FDG)-positron emission tomography (PET) combined with X-ray computed tomography (CT) [9] , [10] , [11] . We used 18F-FDG with micro PET/CT that can be used in rodents to characterize the activity of BBR-treated BAT in vivo . The combination of CT and PET images ( Fig. 2h ) clearly showed that the PET signal was detected higher in the interscapular position of the BBR-treated mice. The calculation results of the standard uptake values showed that BBR has a greater capacity to increase the activity of BAT in drug-treated animals ( Fig. 2i ). Other anatomical sites (indicated with grey triangle) appear to be positive after BBR treatment in PET. Non-BAT-positive absorption may belong to the muscle including skeletal muscle, cardiac muscle, muscle around the backbone and neck by checking the position in CT. Except the location by CT method, the below reasons should be considered. In our study, glucose tolerance test ( Fig. 1d ) and ITT ( Fig. 1g ) show that BBR ameliorates glucose tolerance. And it is worthy of noticing that BBR can stimulate glucose transporter 4 translocation, leading to glucose uptake in skeletal muscle, cardiomyocytes and muscle cell lines [17] , [18] , [19] . BBR promotes thermogenic programme in BAT Consistent with the reduction in body weight, the db/db mice by BBR treatment had smaller brown adipocytes, in which the size of lipid droplets was reduced ( Fig. 3a ), and they accumulated substantially less lipids in the brown fat ( Fig. 3b ). 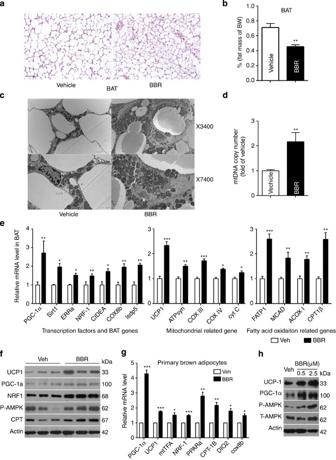Figure 3: Increased thermogenic programme in brown adipose tissue by BBR. (a,b) Representative haematoxylin and eosin staining from interscaptular BAT sections (a) and ratio of BAT to body weight in db/db mice treated with vehicle or BBR (b) (n=5). Ina, original magnification, × 200. Scale bar, 100 μm. (c) Mitochondrial density. Representative transmission electronic microscopy images from BAT of db/db mice treated with vehicle or BBR. Scale bar, 10,000 nm in original magnification × 3,400 and 2,000 nm in magnification × 7,400. (d) MtDNA copy number of BAT from BBR-treated and nontreated db/db mice (n=5). (e) Gene expression profiles in BAT. Db/db mice were treated as described in experimental procedure. Real-time PCR analysis of thermogenic and related gene expression is shown (n=5–7). (f) Representative western blots showing the key protein changes in BAT after BBR treatment. (g,h) Fractionated and differentiated primary BAT adipocytes were treated with 2.5 μM BBR for 24 h. Thermogenic gene expression profile after BBR treatment is shown ing, and representative western blot results of the protein expression level is shown inh. Values represent mean±s.e.m. Error bars represent s.e.m., and significant differences compared with vehicle controls are indicated by *P≪0.05, **P≪0.01 and ***P≪0.001 (assessed by Student'st-test). As shown in Figure 3c , the number of mitochondria was increased as observed by means of transmission electronic microscopy after BBR treatment and quantified by mitochondrial DNA (mtDNA) copy number ( Fig. 3d ). Figure 3: Increased thermogenic programme in brown adipose tissue by BBR. ( a , b ) Representative haematoxylin and eosin staining from interscaptular BAT sections ( a ) and ratio of BAT to body weight in db/db mice treated with vehicle or BBR ( b ) ( n =5). In a , original magnification, × 200. Scale bar, 100 μm. ( c ) Mitochondrial density. Representative transmission electronic microscopy images from BAT of db/db mice treated with vehicle or BBR. Scale bar, 10,000 nm in original magnification × 3,400 and 2,000 nm in magnification × 7,400. ( d ) MtDNA copy number of BAT from BBR-treated and nontreated db/db mice ( n =5). ( e ) Gene expression profiles in BAT. Db/db mice were treated as described in experimental procedure. Real-time PCR analysis of thermogenic and related gene expression is shown ( n =5–7). ( f ) Representative western blots showing the key protein changes in BAT after BBR treatment. ( g , h ) Fractionated and differentiated primary BAT adipocytes were treated with 2.5 μM BBR for 24 h. Thermogenic gene expression profile after BBR treatment is shown in g , and representative western blot results of the protein expression level is shown in h . Values represent mean±s.e.m. Error bars represent s.e.m., and significant differences compared with vehicle controls are indicated by * P ≪ 0.05, ** P ≪ 0.01 and *** P ≪ 0.001 (assessed by Student's t -test). Full size image BBR treatment induced the activation of a network of genes controlling energy expenditure and thermogenic programme in BAT ( Fig. 3e ). The expression of several transcription factors, including PGC-1α, estrogen-related receptor-α and nuclear respiratory factor 1, was strongly activated in the BAT of BBR-treated animals. The expression of the UCP1 and other classical BAT marker genes, such as CIDEA, COX8b and lsdp5, were strongly induced. The expression of genes controlling fatty acid oxidation (FAO) and components of the mitochondrial electron transport chain were enhanced. Western blot analysis indicated that UCP1, PGC-1α, phosphorylation of AMPK and other important proteins expression were enhanced by BBR treatment ( Fig. 3f ). Fractionated and differentiated primary BAT adipocytes were treated with BBR and the patterns of thermogenic gene expression were assessed. The messenger RNA (mRNA) and protein expression of known BAT markers were robustly increased to a high level in the BBR-treated group ( Fig. 3g,h ). These lines of evidence suggest that BBR could function as an activator of thermogenic programming thereby increasing the activity of the BAT. BBR induces browning of inguinal WAT The reduced WAT mass was associated with smaller adipocyte size ( Fig. 4a ), a feature that correlates with leanness and insulin sensitivity. BBR increased the mitochondrial biogenesis as judged by transmission electronic microscopy detection and mtDNA copy number ( Fig. 4b,c ). 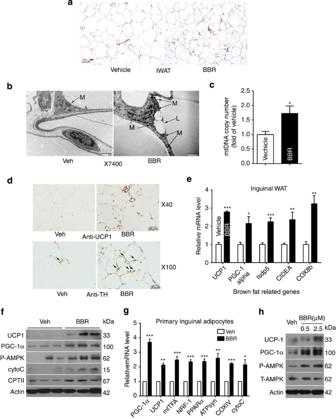Figure 4: Browning of inguinal adipose tissue and activation of a thermogenic programme by BBR. (a) Representative haematoxylin and eosin staining from IWAT sections of db/db mice after 4 weeks of BBR treatment. Original magnification, × 200. Scale bar, 100 μm. (b) Representative electron microscopy micrographs determined in IWAT of vehicle and drug-treated mice. L, lipid droplet; M, mitochondria; Original magnification, × 7400. Scale bar, 2,000 nm. (c) MtDNA copy number of IWAT from BBR or vehicle-treated db/db mice (n=5). (d) Immunohistochemistry for UCP1 protein (brown stain) (upper panel) and TH (lower panel) in IWAT sections of db/db mice treated with vehicle and BBR. (e) BBR induces brown/brite-typical gene expression in IWAT. Real-time PCR analysis of thermogenic gene expression is shown (n=4–6). (f) Representative western blots showing the key protein changes in IWAT. (g) Thermogenic-related gene expression profile in primary IWAT adipocytes after BBR treatment. Primary adipocytes were sourced from IWAT and differentiated as described in ‘Methods’, then treated with 2.5 μM BBR for 12 h. (h) Representative western blots showing the protein expression levels in primary IWAT adipocytes treated with vehicle or BBR. Cells were treated with drug for 24 h. Values represent mean±s.e.m. Error bars represent s.e.m., and significant differences compared with vehicle controls are indicated by *P≪0.05, **P≪0.01 and ***P≪0.001 (assessed by Student'st-test). Figure 4: Browning of inguinal adipose tissue and activation of a thermogenic programme by BBR. ( a ) Representative haematoxylin and eosin staining from IWAT sections of db/db mice after 4 weeks of BBR treatment. Original magnification, × 200. Scale bar, 100 μm. ( b ) Representative electron microscopy micrographs determined in IWAT of vehicle and drug-treated mice. L, lipid droplet; M, mitochondria; Original magnification, × 7400. Scale bar, 2,000 nm. ( c ) MtDNA copy number of IWAT from BBR or vehicle-treated db/db mice ( n =5). ( d ) Immunohistochemistry for UCP1 protein (brown stain) (upper panel) and TH (lower panel) in IWAT sections of db/db mice treated with vehicle and BBR. ( e ) BBR induces brown/brite-typical gene expression in IWAT. Real-time PCR analysis of thermogenic gene expression is shown ( n =4–6). ( f ) Representative western blots showing the key protein changes in IWAT. ( g ) Thermogenic-related gene expression profile in primary IWAT adipocytes after BBR treatment. Primary adipocytes were sourced from IWAT and differentiated as described in ‘Methods’, then treated with 2.5 μM BBR for 12 h. ( h ) Representative western blots showing the protein expression levels in primary IWAT adipocytes treated with vehicle or BBR. Cells were treated with drug for 24 h. Values represent mean±s.e.m. Error bars represent s.e.m., and significant differences compared with vehicle controls are indicated by * P ≪ 0.05, ** P ≪ 0.01 and *** P ≪ 0.001 (assessed by Student's t -test). Full size image As shown in Fig. 4d (upper panel), by performing UCP1 immunohistochemistry, the inguinal WAT (IWAT) of BBR-treated mice was accompanied by a profound morphological transformation towards a BAT-like phenotype, which was observed in numerous clusters of UCP1-expressing multilocular adipocytes under basal conditions. We also quantified sympathetic input to adipose tissue after BBR treatment because thermogenesis is rigorously controlled by the sympathetic nervous system [20] . Notably, we observed a dramatic increase in the expression of tyrosine hydroxylase (TH) in both BAT and IWAT after long term treatment of BBR in wild-type or db/db mice ( Supplementary Figs 3j,k and 4a,b ). Moreover, staining for TH was significantly increased in IWAT of BBR-treated db/db mice ( Fig. 4d , lower panel), suggesting that BBR could augment the sympathetic outflow to IWAT, which might contribute to the BBR effect in browning of IWAT. BBR induced strong expression of UCP1 in the mRNA and the protein ( Fig. 4e,f ). Markers of brown adipocytes, such as PGC-1α, CIDEA, Cox8b and lsdp5, were also significantly increased in IWAT of BBR group ( Fig. 4e ). A much greater induction of transcription factors, thermogenic and FAO gene expression, occurred in the IWAT of the BBR group ( Supplementary Fig. 4c ). Immunoblotting analysis shows that IWAT from the BBR group expressed higher levels of specific BAT proteins such as UCP1 and PGC-1α ( Fig. 4f ). Upregulation of the protein levels of Cyto C and CPT, and phosphorylation of AMPK were also observed ( Fig. 4f ). To investigate whether these alterations in gene expression were mediated by a direct effect, fractionated and differentiated primary IWAT adipocytes were treated with BBR. We observed a strong activation in BAT marker genes (PGC-1α and UCP1), transcription factors (PPARα, nuclear respiratory factor 1 and mTFA) and mitochondrial biogenesis (ATPsyn, COXIV and Cyto C ) (Fig. 4g ). Protein levels of PGC-1α and UCP1 and the phosphorylation of AMPK were simultaneously upregulated by BBR in primary IWAT adipocytes ( Fig. 4h ). Consistent with the data in db/db mice, in wild-type mice, BBR could reduce the body weight gain by increasing energy expenditure and activating a thermogenic programme ( Fig. 6a,c,d,f,h ; Supplementary Fig. 3a–k ). Figure 6: Thermoneutral conditions block the thermogenic programme induced by BBR administration. 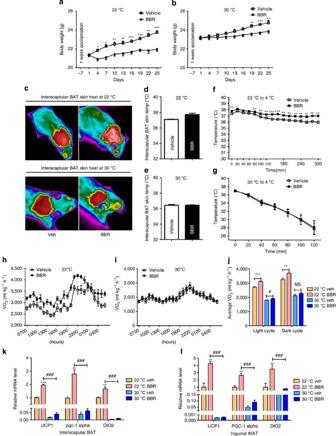Figure 6: Thermoneutral conditions block the thermogenic programme induced by BBR administration. (a,b) Body weight of wild type (WT) mice treated with vehicle or BBR and housed at 22 °C (a) or 30 °C, respectively, (b) every 3 days (n=8). (c–e) Representative infrared thermal images (c) and quantification of temperature of the skin surrounding interscapular BAT in WT mice treated with vehicle or BBR and housed at 22 °C (d) or 30 °C, respectively (e); (f,g) Core body temperature of vehicle and BBR-treated mice during cold challenge after being housed at 22 °C (f) or 30 °C (g) for 4 weeks (n=8). (h–j) Oxygen consumption (VO2) in vehicle and BBR-treated mice at different environmental temperatures, at 22 °C (h) or 30 °C (i); The adjacent bar graphs represent the average comparison of different groups (j) (n=6–7). (k,l) Quantitative reverse transcriptase–PCR analysis of thermogenic genes in interscaptular BAT (k) and inguinal WAT (l) of WT mice treated with or without BBR housed at different environmental temperatures (n=5). Values represent mean±s.e.m.. Error bars represent s.e.m., and significant differences compared with vehicle controls are indicated by *P≪0.05, **P≪0.01 and ***P≪0.001 (Student'st-test); significant differences compared with BBR-treated group in 30 °C are indicated by#P≪0.05,##P≪0.01 and###P≪0.001 (Student'st-test). ( a , b ) Body weight of wild type (WT) mice treated with vehicle or BBR and housed at 22 °C ( a ) or 30 °C, respectively, ( b ) every 3 days ( n =8). ( c – e ) Representative infrared thermal images ( c ) and quantification of temperature of the skin surrounding interscapular BAT in WT mice treated with vehicle or BBR and housed at 22 °C ( d ) or 30 °C, respectively ( e ); ( f , g ) Core body temperature of vehicle and BBR-treated mice during cold challenge after being housed at 22 °C ( f ) or 30 °C ( g ) for 4 weeks ( n =8). ( h – j ) Oxygen consumption (VO2) in vehicle and BBR-treated mice at different environmental temperatures, at 22 °C ( h ) or 30 °C ( i ); The adjacent bar graphs represent the average comparison of different groups ( j ) ( n =6–7). ( k , l ) Quantitative reverse transcriptase–PCR analysis of thermogenic genes in interscaptular BAT ( k ) and inguinal WAT ( l ) of WT mice treated with or without BBR housed at different environmental temperatures ( n =5). Values represent mean±s.e.m.. Error bars represent s.e.m., and significant differences compared with vehicle controls are indicated by * P ≪ 0.05, ** P ≪ 0.01 and *** P ≪ 0.001 (Student's t -test); significant differences compared with BBR-treated group in 30 °C are indicated by # P ≪ 0.05, ## P ≪ 0.01 and ### P ≪ 0.001 (Student's t -test). Full size image BBR does not induce brown-like adipocyte in EWAT There was a significant increase in the thermogenic gene expression levels ( Fig. 5b,c ) but morphological brown-like adipocyte was not seen in the EWAT (epididymal WAT), except the smaller adipocyte size ( Fig. 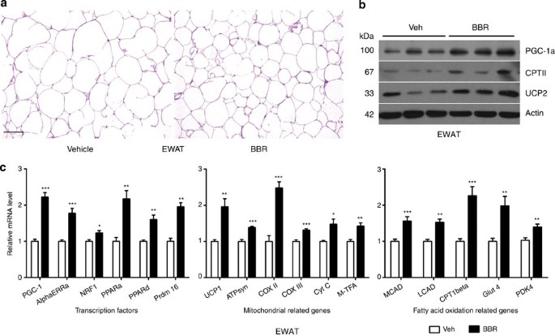5a ) after BBR treatment. Figure 5: BBR does not induce morphological brown-like adipocyte in EWAT. (a) Representative haematoxylin and eosin staining of EWAT histology after 4 weeks of BBR administration. original magnification, × 200. Scale bar, 100 μm. (b) Representative western blots showing the key protein changes in EWAT. (c) Gene expression profile in EWAT. Values are expressed relative to the housekeeping gene (n=5–7). Values represent mean±s.e.m. Error bars represent s.e.m., and significant differences compared with vehicle controls are indicated by *P≪0.05, **P≪0.01 and ***P≪0.001 (assessed by Student'st-test). Figure 5: BBR does not induce morphological brown-like adipocyte in EWAT. ( a ) Representative haematoxylin and eosin staining of EWAT histology after 4 weeks of BBR administration. original magnification, × 200. Scale bar, 100 μm. ( b ) Representative western blots showing the key protein changes in EWAT. ( c ) Gene expression profile in EWAT. Values are expressed relative to the housekeeping gene ( n =5–7). Values represent mean±s.e.m. Error bars represent s.e.m., and significant differences compared with vehicle controls are indicated by * P ≪ 0.05, ** P ≪ 0.01 and *** P ≪ 0.001 (assessed by Student's t -test). Full size image Thermoneutrality blocks thermogenic program induced by BBR Thermoneutral conditions where mice no longer require thermogenesis to maintain body temperature can functionally downregulate the activity of BAT [21] . Feeding at 30 °C (thermoneutrality for mice) resulted in significantly more weight gain than mice housed at 22 °C, which is consistent with previous report [21] . Wild-type mice treated with BBR had a significant less body weight reduction at 30 °C than the animals treated at 22 °C ( Fig. 6a,b ). BBR-treated mice at 30 °C lost the ability to increase core body temperature ( Supplementary Fig. 5a ) and interscaptular BAT skin temperature ( Fig. 6c,e ) when compared with the corresponding group at 22 °C ( Supplementary Fig. 3b , and Fig. 6c,d ), as determined by rectal temperature and infrared imaging of heat intensity. We assessed the metabolic rates by measuring the VO2. At 22 °C, BBR-treated mice showed striking higher oxygen consumption than vehicle group ( Fig. 6h ). When fed at 30 °C, both vehicle and BBR-treated mice showed marked decrease in VO2 ( Fig. 6i,j ). CLAMS result clearly show that thermoneutrality could prevent the contribution of BBR-induced BAT activity to metabolic rate. We further evaluated the cold tolerance ability of mice housed at different temperature conditions, treated with or without BBR. As shown in Figure 6f,g , vehicle-treated mice fed at 22 °C were able to maintain an average core temperature >36 °C for 5 h during cold challenge. BBR-treated mice could maintain higher temperature. Compared with mice acclimated at 22 °C, after thermoneutral conditions feeding, the core temperature of vehicle-treated mice dropped drastically during the cold challenge, BBR group also failed to maintain core temperature, suggesting the indispensable role of active BAT in BBR-increased thermogenic programme. In accordance with above findings, mRNA expression of UCP1, PGC-1α and type 2 deiodinase (DIO2), which is required for uncoupled respiration and thermogenic programme in brown and beige adipocytes, decreased markedly in BAT and IWAT of mice after 30 °C feeding ( Fig. 6k,l ). At thermoneutral condition, BBR could only increase slightly UCP1, DIO2 and PGC-1α expression in mice. BBR regulates UCP1 transcription through AMPK/PGC-1α To elucidate the mechanism of increased browning in IWAT and UCP1 activation, we used differentiated multipotent C3H10T1/2 adipocytes as a cell model. We stained differentiated C3H10T1/2 adipocytes with UCP1 antibody and noted strong staining in the cytoplasm of the BBR group ( Fig. 7a ), which was further verified by immunoblotting ( Fig. 7b ). We stained adipocytes with MitoTracker Red, which is a red-fluorescent dye that stains mitochondrial mass. We found significantly strong Red stain in the cytoplasm of BBR-treated cells ( Fig. 7a ), which means more mitochondrial mass. The mitochondrial copy number was increased by BBR ( Fig. 7c ). We detected mitochondrial activity using a citrate synthase assay, which measures the rate-limiting step of the tricarboxylic acid cycle. Citrate synthase activities were significantly increased in the BBR-group ( Fig. 7d ). 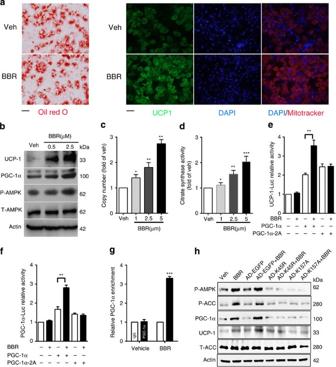Figure 7: BBR-regulated UCP1 expression is AMPK-dependent and involves PGC-1α recruitment. (a) C3H10T1/2 cells were fixed after treatment, then subjected to staining for mitotracker Red, UCP1, and 4',6-diamidino-2-phenylindole (right panel), subsequently to oil red O staining (left panel). Original magnification, × 400. Scale bar, 50 μm. (b) UCP1 and other related protein expression in C3H10T1/2 adipocytes treated with vehicle and BBR (0.5 μM and 2.5 μM, respectively). (c) MtDNA copy number was detected in C3H10T1/2 adipocytes after stimulating with BBR. (d) Citrate synthase activity was measured in C3H10T1/2 adipocytes after a 24 h treatment by BBR. (e,f) HEK293 cells were transfected with an UCP1 construct (UCP1-Luc) (e) and a PGC-1α luciferase promoter construct (PGC-1α-Luc) (f) followed by stimulation (12 h) with BBR. Normalized luciferase activities are shown as fold change. (g) PGC-1α recruitment to the UCP1 promoter region in BBR-treated C3H10T1/2 adipocytes analyzed by ChIP. Fold enrichment are given.n=5 or 6 per condition. (h) C3H10T1/2 adipocytes were infected with adenoviruses encoding enhanced GFP (EGFP), dominant negative forms of AMPK, K45R (α2) and K157A (α1). After BBR treatment, total lysates were analyzed. Values represent mean±s.e.m. Error bars represent s.e.m. Bar graphs represent samples from at least three independent tests, and significant differences compared with vehicle controls are indicated by *P≪0.05, **P≪0.01 and ***P≪0.001 (Student'st-test). Figure 7: BBR-regulated UCP1 expression is AMPK-dependent and involves PGC-1α recruitment. ( a ) C3H10T1/2 cells were fixed after treatment, then subjected to staining for mitotracker Red, UCP1, and 4',6-diamidino-2-phenylindole (right panel), subsequently to oil red O staining (left panel). Original magnification, × 400. Scale bar, 50 μm. ( b ) UCP1 and other related protein expression in C3H10T1/2 adipocytes treated with vehicle and BBR (0.5 μM and 2.5 μM, respectively). ( c ) MtDNA copy number was detected in C3H10T1/2 adipocytes after stimulating with BBR. ( d ) Citrate synthase activity was measured in C3H10T1/2 adipocytes after a 24 h treatment by BBR. ( e , f ) HEK293 cells were transfected with an UCP1 construct (UCP1-Luc) ( e ) and a PGC-1α luciferase promoter construct (PGC-1α-Luc) ( f ) followed by stimulation (12 h) with BBR. Normalized luciferase activities are shown as fold change. ( g ) PGC-1α recruitment to the UCP1 promoter region in BBR-treated C3H10T1/2 adipocytes analyzed by ChIP. Fold enrichment are given. n =5 or 6 per condition. ( h ) C3H10T1/2 adipocytes were infected with adenoviruses encoding enhanced GFP (EGFP), dominant negative forms of AMPK, K45R (α2) and K157A (α1). After BBR treatment, total lysates were analyzed. Values represent mean±s.e.m. Error bars represent s.e.m. Bar graphs represent samples from at least three independent tests, and significant differences compared with vehicle controls are indicated by * P ≪ 0.05, ** P ≪ 0.01 and *** P ≪ 0.001 (Student's t -test). Full size image PGC-1α is a critical transcriptional coactivator that induces UCP1 expression [22] . We investigated the UCP1 promoter because this promoter contains a well-defined PGC-1α binding site that may underlie the induction of UCP1 (ref. 23 ). We also tried the PGC-1α promoter because PGC-1α is involved in the induction of the PGC-1α gene in a feed-forward loop [24] . BBR treatment significantly increased the UCP1 and PGC-1α promoter reporter activities only when PGC-1α plasmid was present, which indicates that PGC-1α was dispensable in BBR’s pharmacological effect ( Fig. 7e,f ). We used chromatin immunoprecipitation (ChIP) to study whether PGC-1α can be recruited to the UCP1 promoter region in C3H10T1/2 cells. A weak PGC-1α signal was present at the UCP1 promoter under basal conditions, and the signal increased robustly after BBR stimulation. BBR stimulation enriched PGC-1α occupancy at the UCP1 promoter region by more than threefold ( Fig. 7g ) when compared with the control immunoglobulin-G (IgG) group. BBR administration enhanced phosphorylation of AMPK in vivo and in vitro ( Figs 3f,h , 4f,h and 7b ). In C3H10T1/2 cells, we blocked the AMPK activity with adenovirus-carrying dominant-negative AMPKs, which almost prevent the total increased expression in PGC-1α and UCP1 that were originally induced by BBR ( Fig. 7h ). Overexpression of the constitutively active PGC-1α 2A (T177A/S538A) mutant, where the two AMPK phosphorylation sites are mutated, caused the promoter luciferase activity to not be further enhanced by BBR ( Fig. 7e,f ). Collectively, our data suggested that BBR could activate AMPK and recruit PGC-1α to the UCP1 promoter, thus inducing UCP1 expression. AMPK in VMH are not necessary for BBR Treatment of BBR in db/db mice showed a reduction in food intake ( Fig. 8a ). Consistent with the hypophagic state induced by BBR, mRNA expression of proopiomelanocortin was increased ( Fig. 8b ). We also observed that 4 weeks BBR treatment decreased phosphorylation levels of AMPK and ACC in hypothalamus ( Fig. 8c ). 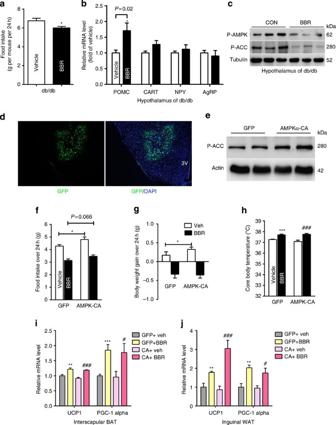Figure 8: AMPK in the VMH is not necessary for activation of the thermogenic programme by BBR. (a) Average daily food intake in vehicle and BBR-treated db/db mice (n=5–6). (b) Hypothalamic expression of neuropeptides after 4 weeks of treatment by vehicle and BBR in db/db mice. The mRNA levels were determined by quantitative reverse transcriptase–PCR (n=5–6). (c) Immunoblots of hypothalamic pAMPK and pACC in hypothalamus of vehicle and BBR-treated db/db mice. (d) Localization of stereotaxically delivered GFP-expressing viruses targeted to the VMH as detailed in the Methods section. (e) Western blot validation of protein levels of pACC of mice stereotaxically injected with adenoviruses encoding GFP and AMPKα-CA. (f–h) Daily food intake (f), body weight change over 24 h (g) and core body temperature (h) of mice stereotaxically targeted with GFP or AMPKα-CA adenoviruses and then treated with vehicle or BBR for 3 days. (i,j) mRNA expression of UCP1 and PGC-1α in interscapular BAT (i) and inguinal WAT (j) of mice stereotaxically treated with GFP or AMPKα-CA adenoviruses and treated with vehicle or BBR for 3 days. Values represent mean±s.e.m. *P≪0.05, **P≪0.01 and ***P≪0.001 (assessed by Student'st-test), Ad-GFP BBR group versus Ad-GFP vehicle group;#P≪0.05,##P≪0.01 and###P≪0.001 (assessed by Student'st-test), Ad-AMPKα-CA BBR group versus Ad-AMPKα-CA vehicle group. Figure 8: AMPK in the VMH is not necessary for activation of the thermogenic programme by BBR. ( a ) Average daily food intake in vehicle and BBR-treated db/db mice ( n =5–6). ( b ) Hypothalamic expression of neuropeptides after 4 weeks of treatment by vehicle and BBR in db/db mice. The mRNA levels were determined by quantitative reverse transcriptase–PCR ( n =5–6). ( c ) Immunoblots of hypothalamic pAMPK and pACC in hypothalamus of vehicle and BBR-treated db/db mice. ( d ) Localization of stereotaxically delivered GFP-expressing viruses targeted to the VMH as detailed in the Methods section. ( e ) Western blot validation of protein levels of pACC of mice stereotaxically injected with adenoviruses encoding GFP and AMPKα-CA. ( f – h ) Daily food intake ( f ), body weight change over 24 h ( g ) and core body temperature (h) of mice stereotaxically targeted with GFP or AMPKα-CA adenoviruses and then treated with vehicle or BBR for 3 days. ( i , j ) mRNA expression of UCP1 and PGC-1α in interscapular BAT ( i ) and inguinal WAT ( j ) of mice stereotaxically treated with GFP or AMPKα-CA adenoviruses and treated with vehicle or BBR for 3 days. Values represent mean±s.e.m. * P ≪ 0.05, ** P ≪ 0.01 and *** P ≪ 0.001 (assessed by Student's t -test), Ad-GFP BBR group versus Ad-GFP vehicle group; # P ≪ 0.05, ## P ≪ 0.01 and ### P ≪ 0.001 (assessed by Student's t -test), Ad-AMPKα-CA BBR group versus Ad-AMPKα-CA vehicle group. Full size image To elucidate the contribution of central AMPK activity in BBR-induced thermogenic programme, adenovirus encoding AMPKα constitutive active (AMPKα-CA) and null green fluorescent protein (GFP) control were injected stereotaxically into ventromedial nucleus of the hypothalamus (VMH) of C57 mice. VMH was chosen as the injection site because evidences demonstrated that selective modulation of AMPK activity in hypothalamus, more specifically in the VMH, might be a useful strategy to treat disorders in energy homoeostasis [25] , [26] , [27] . Correct VMH adenoviral delivery was assessed by GFP immunofluorescence detection and hypothalamic protein levels of pACC ( Fig. 8d,e ). Consistent with previous report [25] , mice injected with AMPKα-CA ate more food and gained more body weight compared with the Ad-GFP group ( Fig. 8f,g ). Although administration of AMPKα-CA had the potential to block the BBR effect on food intake, AMPKα-CA failed to reverse the decrease in body weight after BBR treatment ( Fig. 8f,g ). As shown in Fig. 8h–j , mice overexpression of AMPKα-CA in the VMH was also associated with a reduction in expression of UCP1 and PGC-1α and 0.2 °C drop in core body temperature. BBR still had a marked activation on the above features in the presence of AMPKα-CA. Combined with the above data, we conclude that AMPK in hypothalamus, at least in VMH, was not involved in the BBR’s effect on the thermogenic programme and body weight. Targeting energy expenditure represents an attractive concept for combating obesity [2] . Promoting thermogenic capacity in BAT or obtaining BAT-like characteristics in WAT might be a therapeutic strategy for treating obesity and its complications [28] , [29] . The beneficial effects of BBR on metabolic improvement have evoked a substantial interest in the compound as a potential treatment for obesity and diseases such as diabetes. Our data support a clear function of BBR in regulating energy expenditure by initiating a thermogenic programme. Brown fat is believed to play a thermogenic role and the uptake of FDG within brown fat tissue is well-described on 18F-FDG-PET [30] . To characterize the activity of brown fat tissue in vivo , we conducted a micro PET-CT detection that can be applied in rodents. PET scanning combined with CT location detected a more extensive signal in BAT of mice in the BBR-treated group. These results indicate that BBR-treated brown fat cells function as a sink for active glucose disposal. The BBR treated-mice were resistant to cold exposure, indicating the effects of BBR on the regulation of BAT thermogenesis, which is consistent with the result of micro PET/CT. Given the ability of BAT to dissipate heat from stored chemical energy and thus counteract obesity, we are optimistic that BBR can be used to drive the activity in the brown fat in a therapeutic view. At subthermoneutral environmental temperatures (18–22 °C), extra thermogenesis is needed irrespective of its origin [21] , [31] . Thermoneutral condition feeding, where mice no longer require thermogenesis to maintain body temperature, can functionally downregulate the activity of BAT, which helped us elucidating the role of BAT in the BBR’s pharmacological effect. BBR-treated mice that were fed at 30 °C failed to increase core body and interscaptular BAT skin temperature. After feeding at thermoneutral condition, BBR-treated mice lost its thermogenic capacity, as the dramatically reduced core body temperature and oxygen consumption in these mice are evident. A particular feature of thermoneutral experiments is that administration of BBR still had a weak effect on body weight compared with vehicle-treated animals. A possible explanation is that mice still maintained low BAT activity even under thermoneutrality. BBR has a slight effect on the remaining active BAT, evidenced by the fact that BBR increased the expression of genes related with FAO in the basal state ( Supplementary Fig. 5b,c ). On the other hand, we calculated the oxygen consumption under thermoneutrality condition. Although there is no difference between BBR and vehicle group over a whole day ( P =0.12) and at dark cycle ( P =0.25), at light cycle BBR still has a slightly higher oxygen consumption than vehicle group (Veh versus BBR, 1792.228 versus 1905.994 ml kg −1 h −1 , P =0.03) ( Fig. 6j ). Altogether, these results indicated that functional BAT plays a key role in the BBR’s effect on energy expenditure and thermogenic programme. Our data demonstrated that BBR could induce the thermogenic gene expression and augmentation of a brown fat-like phenotype in subcutaneous WATs and primary cells. In BBR-treated mice, the enhanced fat oxidation might generate a proton gradient in mitochondria, which can subsequently be eliminated through UCP1-mediated uncoupling as heat. Since BBR increased the UCP1 expression and mitochondrial mass in both BAT and IWAT, the increased energy expenditure caused by BBR should possibly involve the browned WAT in part, in spite of the difficulty to measure it directly with the existing method . It is clear that there are two distinct types of brown adipose cells, one of them is the classical brown fat cell that arises from a myf5, muscle-like cell lineage [32] , [33] . This is exemplified by the interscapular BAT deposit and the perirenal BAT deposit, a deposit that contains a mixture of classical brown and white adipocytes [32] , [34] . UCP1-positive brown fat-like cells can also emerge in most WAT deposits upon various stimuli, such as prolonged cold exposure or β-adrenergic receptor activation [35] , [36] . These cells, which are not derived from a myf5-positive lineage, are designated beige or brite cells [37] , [38] . This process is characterized by the appearance of UCP1-positive multilocular adipocytes that serve to increase the thermogenic capacity of the organism. It has been reported that BBR inhibits the differentiation of 3T3-L1 preadipocytes, induced by classic differentiation medium, and suppresses the mitotic clonal expansion of 3T3-L1 preadipocytes in a time and dose-dependent manner through inhibition of the PPARγ pathway [39] . Our results suggest that differentiated primary adipocytes and C3H10T1/2 cells can be stimulated by BBR to express more UCP1 protein, thus BBR seems to drive a white to brown switch in the IWAT through direct transformation of the adult cells rather than the differentiation of preadipocytes. Transdifferentiation is a process by which a mature differentiated cell transforms into a new phenotype with a different morphology and physiology without undergoing dedifferentiation [40] . White-to-brown transdifferentiation, in which britening occurs through a direct interconversion of a white adipocyte into a brown adipocyte phenotype, is of great interest because of its potential use in curbing obesity and its related disorders [34] , [41] , [42] , [43] . Several studies support the notion that this process occurs through the direct transformation of adult cells, that is, via physiological reversible transdifferentiation [36] , [44] . Because the exact origin of brite adipocytes remains under debate [45] , [46] , we cannot exclude the effects of BBR on alternative or additional progenitor cell types committed to the brown fat-like cells in vivo . More fate-mapping experiments are needed to resolve this problem. In classic brown fat depots, thermogenesis is tightly regulated by catecholamines secreted by sympathetic nerve endings in BAT [47] . Moreover, the density of brown-like adipocytes in WAT depots is positively correlated with the number of sympathetic nerve fibres [48] . The enrichment of TH in both BAT and WAT after BBR treatment ensures that the tissues can efficiently undergo thermogenesis in response to the activity of the sympathetic nervous system. Our data also suggest that BBR might drive the browning of IWAT under basal condition by potentially augmenting the adrenergic outflow to IWAT. Although UCP1 mRNA was similarly increased in the IWAT and the EWAT, our findings indicate that BBR can drive a programme of brown adipocyte-like formation only in subcutaneous WAT. The propensity to accumulate brite cells might be different between the above two WAT deposits. Although brown adipocytes can be induced in the epididymal deposits of transgenic animals in response to a strong pharmacological β3-adrenergic stimulus [49] , other pathways have shown that the visceral depot is considered less susceptible to acquiring BAT characteristics compared with subcutaneous fat [47] , [50] . BBR appears to induce the expression of many genes associated with the function of the brown/beige adipocytes. PGC-1α is highly expressed in BAT but expressed at low levels in the WAT [51] . The ectopic expression of PGC-1α in white adipocytes induces the acquisition of BAT features, including the expression of mitochondrial and fatty acid-oxidation and thermogenic genes [22] , [52] . Our results supported that PGC-1α might be critical for BBR’s function and is required for the consequent thermogenic effects of BBR. AMPK is a key regulator of energy metabolism and mitochondrial biogenesis [53] , [54] , [55] . The mechanisms by which AMPK modulates energy are not entirely elucidated, but they seem to require PGC-1α, either by increasing its expression [56] or by direct phosphorylation [57] . The two adenovirus-carrying dominant-negative AMPKs significantly and almost completely reduced the effect of BBR on the expression of PGC1-1α and UCP1. Overexpression of a PGC-1α 2A mutant at sites where the original two amino acids can be phosphorylated by AMPK abolished the increased UCP1 and PGC1-1α promoter luciferase activity by BBR, which demonstrates that AMPK might be an important mediator of BBR effects. Our results demonstrated that AMPK played a key role in thermogenic programme induced by BBR. In recent years, studies demonstrate that AMPK is a target for BBR in the regulation of metabolism [13] , [18] . BBR may activate AMPK through increasing AMP/ATP ratio in 3T3-L1 adipocytes and L6 myotubes [58] . BBR can also activate AMPK by inhibiting mitochondrial respiratory complex I in rat muscles [15] . However, there are other reports that show that BBR could exert pharmacological effects in a AMPK-independent manner [59] . For AMPK-induced brown adipocytes within WAT depots, distinct results have been described. It was reported that activation of AMPK using AICAR in rats increases energy expenditure and mitochondrial content but not UCP1 expression in subcutaneous and visceral WAT of male Wistar rats [60] . Another study reported that AICAR treatment induced an accumulation of brown adipocytes in EWAT of mice [61] . Our results showed that BBR could drive the browning of IWAT in db/db mice through AMPK activation. Species differences, duration of treatment, dosage and frequency of injections might explain the different results of these studies. Moreover, to our knowledge there is no report about the browning of WAT on the knockout or transgenic mouse model of AMPK, which could provide a direct proof. Previous studies show that hypothalamic VMH AMPK could be involved in BAT thermogenesis and peripheral browning in WAT [62] , [63] . However, AMPK in hypothalamus at least in VMH was not involved in BBR’s effect, as stereotaxically delivery of adenovirus encoding constitutive active AMPKα could not block weight loss, thermoregulation and increased expression of thermogenic markers in BAT and IWAT induced by BBR. It might be plausible that VMH AMPK was not involved in BBR’s thermogenic effect because BBR still showed robust induction in thermogenic programme in primary brown and white adipocytes. However, we could not exclude the possibility if another nuclei of hypothalamus, such as arcuate or another part of brain, participated in the thermogenic programme induced by BBR, which needs to be studied further. Combined with our work, BBR could activate and expand the thermogenic machinery in vivo to provide a robust defence against obesity. We reveal the molecular target and mechanism by which BBR potently regulated the transcription of UCP1 in brown and white adipocytes through AMPK activation and PGC-1α recruitment. These findings establish an important role for BBR in regulating adipose tissue thermogenesis and white adipose plasticity towards BAT, and we identify BBR as a new potential drug for treating patients with obesity. Chemicals and antibodies BBR was purchased from Sigma-Aldrich (MO, USA). The antibodies used for immunoblotting included anti-UCP1 (Alpha Diagnostic), anti-phospho-AMPK, anti-total AMPK (Cell Signaling), anti-PGC-1 (Millipore), anti-actin (calbiochem) and anti-Cyto C (BD bioscience). All the other chemicals were purchased from Sigma Chemical Co. unless otherwise specified. Cell culture and adenoviral infection Primary white and brown fat stromal vascular and mature fat cells were fractionated by collagenase digestion according to the published methods as described elsewhere [64] , [65] , [66] . C3H10T1/2 cells were obtained from ATCC. Primary stromal vascular cells and C3H10T1/2 were maintained in Dulbecco’s modified Eagle’s medium (DMEM) with 10% foetal bovine serum (FBS; Invitrogen) at 37 °C in a 5% CO 2 environment. Adipocyte differentiation was induced in preadipocyte cultures by treating confluent cells for 48 h in medium containing 10% FBS, 0.5 mM isobutylmethylxanthine, 125 nM indomethacin, 1 μM dexamethasone, 850 nM insulin and 1 nM T3 with 1 μM rosiglitazone (Alexis Biochemicals). After 48 h, the cells were moved to the medium containing 10% FBS, 850 nM insulin and 1 nM T3 with 1 μM rosiglitazone [47] . The plasmids for adenoviruses construction encoding c-Myc-tagged forms of AMPK constitutively active α1 (T172D), dominant-negative α1 (K157A)and α2 (K45R) AMPK (DN-AMPK) [67] were kind gifts from Dr J. Ha (Department of Molecular Biology, Kyung Hee University College of Medicine, Seoul, Korea). C3H10T1/2 adipocytes were used after 48 h of differentiation. The cells were washed with PBS and left for 1 h in serum-free DMEM with 4.5 g l −1 of glucose containing the appropriate amount of viral particles (multiplicity of infection=100 per each virus used, using enhanced GFP as a control to equalize the final viral amount). The media was replaced with fresh differentiation media for additional days before any treatment took place. DMSO was used as the vehicle for different treatments. Animal experiments The animal protocol was reviewed and approved by the Animal Care Committee of the Shanghai Jiao Tong University School of Medicine. Obese C57BLKS/J-Leprdb/Leprdb (db/db) male mice and wild-type mice were purchased from the Model Animal Research Center of Nanjing University. At 9-weeks of age, the mice were housed at 22±2 °C, 55±5% relative humidity and with a 12 h light/dark cycle. Food (Slaccas, Shanghai, China) and water were given ad libitum . BBR was i.p. (5 mg kg −1 per day) injected into the mice for 4 weeks between 0900 and 1000 hours. In thermoneutrality experiments, mice of each group were singly caged and housed at 30 °C, with a 12:12 h light/dark cycle, for the duration of the experiment. Seven days after being acclimatized at 30 °C, BBR and vehicle were administrated for the next 4 weeks. The experiments were not randomized, and the investigators were not blinded to allocation during experiments and outcome assessments. No statistical method was used to predetermine sample size. Metabolic rate and physical activity Oxygen consumption and physical activity were determined for male mice at 11-weeks-of-age using CLAMS (Columbus Instruments) according to the manufacturer’s instructions. The animals were acclimated to the system for 20–24 h, and measurement of VO2 and VCO2 was performed during the next 24 h. The mice were maintained at 24 °C under a 12-h light/dark cycle. Food and water were available ad libitum . Voluntary activity was derived from the x -axis beam breaks monitored every 15 min. Heat production and the RER were calculated as described previously [68] . Histology and immunofluorescence Tissues fixed in 4% paraformaldehyde were sectioned after being paraffin embedded. Multiple sections were prepared and stained with haematoxylin and eosin for general morphological observations. Cells grown on poly-L-lysine (Sigma)-pretreated coverslips were fixed with 4% paraformaldehyde. Immunofluorescence staining was performed according to the standard protocol using the following antibodies and dilutions: UCP1 1:100, MitoTracker Red (Invitrogen) 1:1000. The incubations were performed overnight in a humidified chamber at 4 °C. The secondary antibodies for immunofluorescence staining were purchased from Invitrogen. 4,6-diamidino-2-phenylindole staining was used to mark the cell nuclei. Immunofluorescence staining was performed first and immunofluorescent images were captured. Then slides were immersed in PBS to remove the mounted coverslip and were subjected to oil red O staining. The images were acquired using an Olympus BX51 system. Glucose and ITT A glucose tolerance test was performed in male db/db mice after an overnight fast. The glucose concentrations were measured in blood collected by venous bleeding from the tail vein immediately before and, 15, 30, 45, 60, 90 and 120 min, after a bolus i.p. injection of glucose at 0.75 g kg −1 . An ITT was performed in a 6-h (0800–1400 hours) fasting mice. The glucose concentrations were measured by venous bleeding at 0, 15, 30, 45, 60, 90 and 120 min after an i.p. injection of human insulin (Eli Lilly) at 2 U kg −1 . Cold tolerance test A cold tolerance test was performed in a 12-week-old mice. The animals were then subjected to a cold room (4–8 °C) without access to food or water. The rectal temperature was measured at the indicated time after exposure to the cold. Temperature measurements The body temperature was measured at room temperature at 0900 hours using a rectal probe connected to digital thermometer (BAT-12 Microprobe-Thermometer; Physitemp; NJ, USA). Skin temperature surrounding BAT was recorded with an infrared camera (E60: Compact-Infrared-Thermal-Imaging-Camera; FLIR; West Malling, Kent, UK) and analyzed with a specific software package (FLIR ResearchIR Max 3.4; FLIR; West Malling). We used 6–8 mice per group and for each animal three to four pictures were analyzed. The skin temperature surrounding BAT for one particular animal was calculated as the average temperature recorded by analyzing those pictures. Micro PET/CT PET/CT imaging was performed on an Inveon MM Platform (Siemens Preclinical Solutions, Knoxville, TN, USA) at the Shanghai Jiao-tong University Med-X Ruijin Hospital Micro PET/CT Research Center. Mice were allowed to fast overnight and were lightly anesthetized with isoflurane followed by a tail vein injection of 18F-FDG (150 μCi). Sixty mins after the injection of the radiotracer, the mice were subjected to PET/CT analysis. Inveon Acquisition Workplace (IAW) 1.5.0.28 was used for the scanning process. A 10 min CT X-ray for attenuation correction was scanned with a power of 80 kv and 500 μA and an exposure time of 1,100 ms before the PET scan. Ten-minute static PET scans were acquired, and the images were reconstructed by an OSEM3D algorithm followed by Maximization/Maximum a Posteriori (MAP) or FastMAP provided by IAW. The three-dimensional regions of interest (ROIs) were drawn over the guided CT images, and the tracer uptake was measured using the software of Inveon Research Workplace (IRW) 3.0. Individual quantification of the 18F-FDG uptake in each of the ROIs was calculated. The data for the accumulation of 18F-FDG on micro PET images were expressed as the standard uptake values, which were determined by dividing the relevant ROI concentration by the ratio of the injected activity to the body weight. The data are presented as the mean±s.e.m. Quantitative real-time PCR analysis The total RNA was prepared with the Trizol method (Invitrogen) following the manufacturer’s instructions. Complementary DNA was prepared from 1 μg of RNA using the Reverse Transcription System (Promega). PCR reactions were run in duplicate for each sample and analyzed in the LightCycler 480 Real-Time PCR System (Roche Diagnostics GmbH, Mannheim, Germany). The data were expressed as arbitrary units after normalization to the levels of expression of the internal control actin or 36B4 for each sample. Sequences of the primers used in this study are listed in Supplementary Table 1 . Immunoblotting Homogenized tissue and cells were lysed in RIPA buffer containing protease and phosphatase inhibitors. The protein lysates were separated with SDS–PAGE and electroblotted to polyvinylidene fluoride (Millipore). Electrophoresis supplies were from Bio-Rad Laboratories. The membranes were blocked and incubated with different antibodies, followed by incubation with horseradish peroxidase-conjugated secondary antibodies. Western blot analysis was conducted using enhanced chemiluminescence reagents (Amersham Pharmacia) according to the manufacturer’s protocol. The original scans of immunoblots and antibodies used in this paper are listed in Supplementary Fig. 6 and Supplementary Table 2 . Stereotaxic microinjection of adenoviral expression vectors Male C57BL/6J mice (aged 7–8 weeks) were purchased from Shanghai SLAC laboratory Animal Co., Ltd. (SLAC). Mice were housed in individual cages in a temperature-controlled environment with a 12/12-h light/dark cycle. The mice were given chow diets and water freely before beginning the experiments. Mice were anesthetized and placed in a stereotaxic frame (Kopf Instruments). According to the atlas of the mouse brain, [69] stereotaxic coordinates for intrahypothalamic injection are as follows: Anterior/Posterior axis, 1.30 mm from Bregma to the posterior; Lateral, ±0.5 mm from midline; Depth, 5.70 mm from surface of the skull [28] . Adenoviruses vectors either GFP (2 × 106 p.f.u. μl − , control adenoviruses) or AMPKα constitutively active T172D (AMPKα-CA; 2 × 106 p.f.u. μl −1 ) were delivered at a rate of 40 nl min -1 for 5 min, the pipette was left in place for 5 min and then moved to another side. Correct VMH adenoviral delivery was assessed by injecting Ad-GFP and by immunofluorescence analysis. After 7 days of recovery, BBR and vehicle were administrated by i.p. injection for 3 days. Cell transfection and reporter assays HEK293 cells were transfected with corresponding plasmids for a reporter assay using lipofectamin2000 (Invitrogen). The plasmids for PGC-1α and the PGC-1α2A (T177A/S538A) mutant and the 2-kb PGC-1α ref. 24 reporter were gifts from Professor Bruce M. Spiegelman. UCP1 promoter luciferase reporter constructs were generated based on the study by Pan et al. [23] Twenty-four hours after transfection, the cells were stimulated with BBR as indicated. The cell lysates were harvested after drug administration, and the luciferase activity was measured using the Dual-Luciferase Reporter Assay System (Promega). Firefly luciferase reporter gene measurements were normalized to Renilla luciferase activity Chromatin immunoprecipitation ChIP was performed in BBR versus vehicle-stimulated C3H10T1/2 adipocytes using the EZ-ChIP kit following the manufacturer’s instructions (Millipore), and antibodies to PGC-1α (H-300; Santa Cruz) or normal rabbit IgG (Cell Signaling) were used as a negative control. Differentiated C3H10T1/2 cells were treated with BBR or with vehicle and were fixed with formaldehyde. The DNA was sheared to fragments of 200–1,000 bp by several sonications. The immunoprecipitated DNA was amplified by real-time PCR using primers specific for the mouse UCP1 promoter region. Relative PGC-1α at the UCP1 promoter was determined and normalized to the input DNA. Transmission electron microscopy BAT and IWAT sections were fixed in 2% (vol/vol) glutaraldehyde in 100 mM phosphate buffer, pH 7.2 for 12 h at 4 °C. The sections were then post-fixed in 1% osmium tetroxide, dehydrated in ascending gradations of ethanol and embedded in fresh epoxy resin 618. Ultra-thin sections (60–80 nm) were cut and stained with lead citrate before being examined on the Phillip CM-120 transmission electron microscope. MtDNA content quantification by quantitative real-time PCR Genomic DNA was isolated from WAT and BAT of vehicle-treated mice and BBR-treated mice, respectively. The above tissues were homogenized and digested with Proteinase K overnight in a lysis buffer for DNA extraction by a conventional phenol–chloroform method or by using the DNeasy Blood & Tissue Kit (Qiagen) following the manufacturer’s instructions. The results were calculated from the difference in the threshold cycle (ΔCT) values for mtDNA and nuclear-specific amplification by quantitative real-time PCR. The data are expressed as mtDNA-specific 16S ribosomal RNA normalized to nuclear specific gene hexokinase, which was described in the study by Lagouge et al. [70] Sequences of the primers used in this study are listed in Supplementary Table 1 . Statistical analyses All the data are given as mean±s.e.m. Comparisons between the two groups were assessed by Student’s t -test for independent samples. A P -value ≥0.05 was considered statistically significant. How to cite this article: Zhang, Z. et al. Berberine activates thermogenesis in white and brown adipose tissue. Nat. Commun. 5:5493 doi: 10.1038/ncomms6493 (2014).